Correspondence: Reply to ‘DNA shape is insufficient to explain binding’ 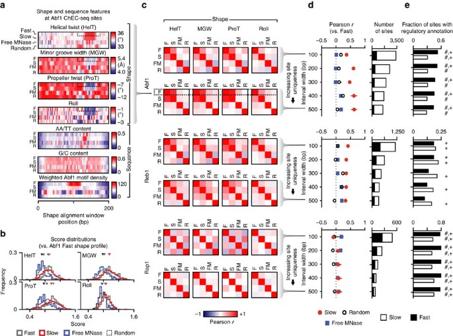Figure 1: Slow ChEC-seq sites have characteristic shapes separate from TF-binding motifs. (a) Average shape and sequence features for unique fast (F) and slow (S) Abf1 sites 500 bp from other ChEC sites compared to free MNase (FM) and random (R) control sites aligned using shape features. Motif density was computed by weighting occurrences based on motif score. (b) Distributions of scores from searching shape vectors using the Abf1 fast site shape profile for fast and slow Abf1 sites (500 bp from other ChEC sites) and free MNase and random control sites; triangles represent the median score for each distribution. The shape profile used for searching is indicated in the dotted boxes ina. (c) Pearson correlations of average DNA helix twist (HelT), minor groove width (MGW), propeller twist (ProT), and roll features for unique fast and slow Abf1, Reb1 and Rap1 sites 100 bp (top) or 500 bp (bottom) from other ChEC sites compared to control sites aligned using shape features. (d) Pearson correlations compared to fast sites of aligned average DNA shape features at a variety of interval widths and the number of sites at each interval width. Error bars represent mean±s.e.m. (e) Proportion of unique sites at a range of overlap interval widths with known or proposed regulatory associations.Pvalues<0.1 under Fisher’s exact test versus FM and R control sites are indicated with ‘#’ and ‘+’, respectively. We defined unique sites such that the intersection of intervals of 100–500 bp widths centred on unique Abf1, Reb1, Rap1 and Free MNase ChEC-seq peak maxima was disjoint. As a null set, we generated 1,500 random intervals from the sacCer3 genome assembly that did not overlap with ChEC-derived peaks. Shape features in 201-bp windows centred on peak maxima were determined as described [4] using the DNAshapeR package [18] . At each interval width for a given TF, sites that did not have overlapping shape alignment windows were selected for alignment. Motif-independent alignment involved comparing each site against every other site within a given class and determining the shift that maximized the cosine similarity. Within a class, all sites were aligned to an internal centroid, defined as the site with the smallest sum of squared cosine similarities versus all other sites. Sites were then shifted relative to the centroid and class-specific average features were computed. Pearson’s r was used to quantify the similarity of average shape features between classes (reported P values are two-tailed) without shifting the average features relative to each other. Given the strong A/T MNase cleavage preference (not shown) in the 5-bp window centred on peak maxima, we excluded these positions from the alignment. Further, because shape readout likely occurs near the TFBS, the largest shift considered was 25 bp and alignment was limited to the 90-bp interval centred at the peak maximum. Parameters used for all site classes including the random and free MNase sites were identical. Shape profiles for Abf1 and Reb1 were defined as the regions in the average fast shape features with the largest information gain relative to shuffled sequences. Score distributions were generated by scoring the aligned fast, slow, free MNase and random sites in the same 90-bp interval used for shape alignment using correlation distance to the shape profile; Mann–Whitney U-tests were performed for pairwise comparisons of the resulting distributions. To determine whether putative TFBSs regulate nearby genes, we assigned them to their closest (≤1 kb) genes and queried YEASTRACT [6] . Source code for these analyses is publicly available ( https://github.com/sivakasinathan/shape_align ). How to cite this article: Kasinathan, S. et al . Correspondence: Reply to ‘DNA shape is insufficient to explain binding’. Nat. Commun. 8, 15644 doi: 10.1038/ncomms15644 (2017). Publisher’s note : Springer Nature remains neutral with regard to jurisdictional claims in published maps and institutional affiliations.